Scalable high-density peptide arrays for comprehensive health monitoring There is an increasing awareness that health care must move from post-symptomatic treatment to presymptomatic intervention. An ideal system would allow regular inexpensive monitoring of health status using circulating antibodies to report on health fluctuations. Recently, we demonstrated that peptide microarrays can do this through antibody signatures (immunosignatures). Unfortunately, printed microarrays are not scalable. Here we demonstrate a platform based on fabricating microarrays (~10 M peptides per slide, 330,000 peptides per assay) on silicon wafers using equipment common to semiconductor manufacturing. The potential of these microarrays for comprehensive health monitoring is verified through the simultaneous detection and classification of six different infectious diseases and six different cancers. Besides diagnostics, these high-density peptide chips have numerous other applications both in health care and elsewhere. Early, presymptomatic detection and treatment of disease often affords a much higher probability of favourable outcome than does intervention at later stages, common with symptomatic presentation (for example, ref. 1 ). This is particularly the case with many chronic diseases such as cancer, where resection at stage 1 often results in an effective cure that is nearly impossible to achieve once metastasis has taken place. In addition, early detection is expected to lower health-care costs [2] . However, moving from a reactive, symptom-based treatment of disease to a proactive, data-based health-maintenance paradigm will almost certainly require the development of very low cost, comprehensive molecular diagnostic tools that are simple to implement and minimally invasive. Current biomarker research has focused on the development of single molecular biomarkers [3] or small panels of biomarkers [4] , and essentially always for one or a small family of diseases. Thus far, this kind of biomarker research has yielded relatively few validated markers, even though a great deal of effort and resources have been expended in their development [5] , [6] , [7] . We recently demonstrated the feasibility of a fundamentally different approach to diagnosis, purposefully aligned with the concept of proactive health monitoring. This approach involves measuring the profile of the circulating antibodies, referred to as an immunosignature. The assay itself requires <1 μl of blood, and the blood can be sent via mail as a drop dried on a piece of filter paper [8] . The blood is diluted with little or no additional processing and incubated with a large array of different non-natural-sequence peptides (reviewed in Sykes et al. [9] ). Our initial platform was an array of 10,000 presynthesized peptides spotted on a glass slide, and we have used this format to characterize immune responses to vaccines [10] , infectious diseases [11] , cancer [12] , [13] , Alzheimer’s Disease [14] and autoimmune disorders [12] . The work on brain cancer [13] was performed as a blinded train/test study, training on a patient cohort taken in 2007 and testing on a cohort from 2010, with 100% accuracy of identification. We have also shown that it is feasible to detect signatures before the onset of symptoms in mouse models [15] and in human pre-pancreatic cancer samples [12] . Importantly, because the peptide sequences are not from any particular proteome, but from non-natural-sequence space, all of the immunosignature diagnoses published and in review to date were carried out with essentially the same array of 10,000 peptides. The biochemical and biophysical features required to create immunosignatures have been studied in detail [16] . The work cited above has been performed using peptides spotted on glass slides. Such arrays are inherently limited by the density of peptides that can be physically spotted, the scalability and reproducibility of fabrication, and ultimately the cost per assay. Many issues arise because of the heterogenic nature of presynthesized peptide chemistry. Ensuring solubility, exact concentration and purity of thousands of peptides stored in liquid buffer is remarkably challenging and affects the ultimate quality of the microarray. The large number of circulating antibodies (~10 9 ) [17] suggest that arrays with more peptides than the current 10 4 would offer better resolution of disease signatures. The most advanced form of spotted arrays has been reported by Frank [18] using the SPOT technology. Peptides are synthesized on spots on filters, the spots individually removed, the peptides released and spotted on glass slides. Densities of 40 features per slide have been obtained [19] . Although the production and utility of low to moderate sized peptide arrays has been demonstrated [20] , [21] , much higher feature densities and more consistent peptide quality should be attainable by using in situ peptide synthesis. In situ synthesis of peptides was first demonstrated more than 20 years ago [22] ; however, to date, the peptide arrays that are commercially available or reported in the literature would not be able to achieve the requirements of low cost, high volume, with well-characterized composition and diagnostic effectiveness that would be needed for a broadly used early diagnostic platform. Recently Price et al. [23] demonstrated the use of photolithography to synthesize peptide arrays on silicon wafers, creating arrays of 9,096 peptides using eight different amino acids. Although that study did not demonstrate scalability, number or complexity of peptides needed for health monitoring using immunosignatures, it and other reports [18] , [22] , [24] , [25] , [26] have shown the potential for peptide array production using the highly refined equipment and techniques of the electronics industry. Using a maskless, light-directed system, Nimblegen-Roche has produced arrays of high density (potentially 2 M per slide) but this system is low volume production. PEPperPRINT Inc. (Heidelberg, Germany) produces peptide arrays using a process based on electrostatic deposition and conjugation of dry amino acids, similar to the method used by laser printers. These arrays are also low volume production and, although they can produce up to 775 peptides per cm 2 , the arrays are tuned more for epitope detection than immunosignaturing [27] . A problem yet to be solved with all in situ systems reported to date is the molecular characterization of the peptides. Most reports qualify the arrays using detection of a few linear epitopes that bind well-characterized, commercially available monoclonal antibodies. However, this says little about chemical purity of the sequences. The lack of direct, in situ chemical analysis remains a major roadblock in the development of high-quality peptide arrays. Here we demonstrate the production of high-density peptide arrays on silicon wafers using scalable manufacturing approaches that lend themselves to low cost and high volume. These arrays have the number of features, quality of peptides and the amino-acid complexity required for immunosignatures. The chemical identity and purity of the in situ synthesis on these arrays is characterized directly by imaging mass spectrometry, using methods we previously developed [28] . Finally, we demonstrate that immunosignatures generated using these arrays can discriminate multiple different infections and cancers from each other with statistical confidence that is as good or better than the printed arrays that have been the basis of our previous work. Quality control of peptide synthesis Specificity of the nine monoclonal antibodies (HA, Ab1, Ab8, Cdc2, DM1A, LNKB2, HSV, 4C1 and A10) to their cognate sequence is high, even in the presence of >330,000 other random-sequence peptides ( Fig. 1a , left panel). Interestingly, each monoclonal antibody tested demonstrates unique behaviour relative to non-cognate peptide sequences [16] . For TP53 Ab1 (AbCam, Preston, MA, USA), for example, there are 209 perfect match epitope sequences (RHSVV) and 98 single-residue mismatch peptides (RHSVG) scattered across each array. We measured the 209 perfect match peptides relative to binding of TP53 Ab1 and obtained a coefficient of variation <5%. We measured a 26-fold difference in average intensity between these 209 perfect match peptides and the 98 single mismatch peptides. As we have previously published, a given monoclonal antibody may exhibit high binding to sequences that are quite divergent from the known epitope [16] . 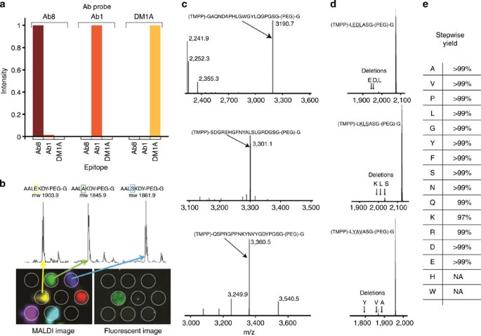Figure 1: Fidelity and stepwise yield ofin situpeptide synthesis. (a) Cognate epitopes for monoclonal antibodies p53Ab8 (epitope: SDLWKL), p53Ab1 (RHSVV) and DM1A (AALEKD) were synthesized 2,163 times as part of the 330,000 feature array. Average binding levels of each monoclonal antibody (Ab probe) with each epitope (nine measurements) are shown and normalized to binding to the cognate epitope. (b) The DM1A epitope and several variants were synthesized in 200-μm features on the same wafer. Both a MALDI image (different colours represent different molecular weights) and a fluorescence image of labelled DM1A Ab binding are shown. MALDI spectra extracted from several of the imaged features over a 160 D mass range are provided. The small peak to the right of the main peak represents incomplete side chain deprotection. (c) MALDI mass spectra from individual 200-μm features in which peptides containing 21 amino acids plus a tris (2,4,6-trimethoxyphenyl)phosphonium-acetyl (TMPP-Ac) group and a 30-atom polyethylene glycol linker were synthesized. (d) A series of 10-mer peptides were synthesized in 200-μm features that differed only in three amino acids (bold and underlined). The full-length peptide and the expected mass for each of the single deletion products of the variable amino acids are shown (marked by arrows). (e) The yields for each amino acid determined from measurements described in part (d). Measurements of multiple peptides containing each amino acid gave s.e.’s of 1% or less. The conditions used to release the peptides from the surface appear to affect the MALDI signals for Trp and His, so yields for these amino acids are not known. Figure 1: Fidelity and stepwise yield of in situ peptide synthesis. ( a ) Cognate epitopes for monoclonal antibodies p53Ab8 (epitope: SDLWKL), p53Ab1 (RHSVV) and DM1A (AALEKD) were synthesized 2,163 times as part of the 330,000 feature array. Average binding levels of each monoclonal antibody (Ab probe) with each epitope (nine measurements) are shown and normalized to binding to the cognate epitope. ( b ) The DM1A epitope and several variants were synthesized in 200-μm features on the same wafer. Both a MALDI image (different colours represent different molecular weights) and a fluorescence image of labelled DM1A Ab binding are shown. MALDI spectra extracted from several of the imaged features over a 160 D mass range are provided. The small peak to the right of the main peak represents incomplete side chain deprotection. ( c ) MALDI mass spectra from individual 200-μm features in which peptides containing 21 amino acids plus a tris (2,4,6-trimethoxyphenyl)phosphonium-acetyl (TMPP-Ac) group and a 30-atom polyethylene glycol linker were synthesized. ( d ) A series of 10-mer peptides were synthesized in 200-μm features that differed only in three amino acids (bold and underlined). The full-length peptide and the expected mass for each of the single deletion products of the variable amino acids are shown (marked by arrows). ( e ) The yields for each amino acid determined from measurements described in part ( d ). Measurements of multiple peptides containing each amino acid gave s.e.’s of 1% or less. The conditions used to release the peptides from the surface appear to affect the MALDI signals for Trp and His, so yields for these amino acids are not known. Full size image While reaction with monoclonal antibodies is the current standard for quality assessment of peptides synthesized in commercial arrays (as shown in Fig. 1a ), this type of analysis does not provide information about the chemical purity or composition of the peptides in each feature, nor does it allow evaluation of the efficiency of individual steps in the process. The chemical purity and yield of synthesis of peptides on the arrays manufactured by HealthTell Inc. (Chandler, AZ, USA) for this study was analysed by generating 200-μm test features on the same wafers as the immunosignature arrays and performing MALDI (matrix-assisted laser desorption ionization) mass spectrometry imaging on those features, after gas phase release of peptides from the surface ( Fig. 1b , left panel). Mass spectra of three of these features, each a variant of the epitope for the monoclonal antibody DM1A, are shown, demonstrating that the appropriate sequences were generated. A fluorescent image of the same array features is also shown ( Fig. 1b , right panel), demonstrating specific binding of the antibody to the cognate sequence (AALEKDY). Figure 1c shows mass spectra of several peptides made with 23 coupling steps, showing that long sequences can effectively be generated. Figure 1d shows a series of spectra from shorter peptides that differed from each other in only three amino acids. Coupling yields of the three variable amino acids were estimated by comparing the ion intensity of the full-length peak with the ion intensity observed at the positions expected for each possible amino-acid deletion (see arrows). The yields shown in Fig. 1e for each amino acid represent the average of results from multiple peptides containing that amino acid. The average yields are at or above those achieved by bead-based peptide synthesis. We were unable to estimate yields for histidine and tryptophan as peptides containing these amino acids appear to be partially oxidized during analysis. However, the monoclonal antibody results from Fig. 1a suggest that both of the amino acids are incorporated, as those epitopes contain both W and H. We conclude that the designated peptides are synthesized in high yield. Immunosignature diagnostic performance The other question in qualifying the system is whether these arrays can reproducibly generate immunosignatures from patients with the same disease. 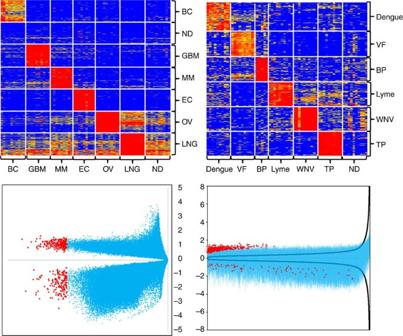Figure 2: Immunosignature performance. Heatmaps (top left and right) indicate groupwise specificity of peptide signals with hierarchical clustering performed on 350 peptides (yaxis) and 60 patients plus 10 controls (xaxis) with Euclidean distance used as the measure of separation. The order of each patient and peptide is calculated from the distance measure using hierarchical clustering. Classification of all samples was 100% accurate using either linear discriminant analysis or support vector machine (SVM) with leave-one-out cross-validation. Top left: serum from six different cancers with 10 patients in each group (BC, breast cancer, GBM,Glioblastoma multiformae, MM, multiple myeloma, EC, oesophageal cancer, OV, ovarian cancer, LNG, lung cancer) was analysed using the 330,000 peptide microarray. The striking stair-step pattern is because of the clustering algorithm alone. Top right: Sera from six different infectious diseases, with 10 patients in each group except BP, with five patients (Dengue, dengue virus, VF,Coccidioides immitis, BP,B. pertussis, Lyme,Borrelia burgdorferi, WNV, West Nile Virus, TP,T. pallidumand healthy donors (ND) were likewise analysed. Each sample set achieved 100% accuracy using SVM as the classifier and leave-one-out cross-validation. Below left: a plot of log10Pvalue (xaxis) versus log2fold-change (yaxis) between 10 randomly selected patients at the time of diagnosis with oesophageal cancer (numerator) and 10 otherwise healthy controls (denominator) displays the distribution of significant peptides and the resulting ratios. In all, 562 peptides withP-val <3 × 10−7are coloured red, yielding a 0.017% false-positive rate. Lower right is a power plot demonstrating the minimum detectable fold-change (delta, black line, calculated using the command power.t.test() in R) along thexaxis. This power plot is reviewed in detail in ref.30. The blue bars (yaxis) represent every peptide’s average log2 ratio between 10 oesophageal cancer patients (numerator) and 10 healthy controls (denominator). The red circles indicate the same peptides as in the graph to the left (P<3 × 10−7). Figure 2 demonstrates this capability. The top left portion of Fig. 2 demonstrates the simultaneous discrimination between six different cancer cohorts (breast cancer, Glioblastoma multiforme , multiple myeloma, oesophageal cancer, ovarian cancer and lung cancer) and healthy normal controls each using sera from 10 different patients. Figure 2 top right demonstrates the discrimination between six different infectious disease cohorts (Dengue fever, Valley fever, Lyme disease, West Nile Virus, Bordetella pertussis (whooping cough) and Treponema palladium (Syphilis) and healthy normal controls, each using sera from 10 different patients (with the exception of B. pertussis with five patients). The peptide intensities for each individual were screened statistically to find the peptides that best represent common reactivity within a disease cohort, with simultaneously low signal in other diseases (GeneSpring 7.3.1, Agilent, Santa Clara, CA, USA). Each peptide feature was selected for both high sensitivity (to detect low copy antibodies) and high specificity (selected peptides should respond to only one disease). A total of 350 peptides (50 per cohort) were selected for the cancer samples ( Fig. 2 , top left) and for the infectious disease samples ( Fig. 2 , top right). More than 50 peptides met the requirements for each condition; however, only the top 50 were used in this analysis. Previous studies indicated information content should peak between 20 and 100 features per disease [16] and the performance of linear classifiers tends to suffer as the total number of features increases [29] . The top 50 informative peptides and important sequence motifs are listed in Supplementary Tables 1 and 2 . As described below (see Analysis), the peptide features that showed common reactivity to each cohort were highly significant statistically. To date, no diagnostic of which we are aware can simultaneously discriminate between six cancers and six infectious diseases using the same platform. Figure 2: Immunosignature performance. Heatmaps (top left and right) indicate groupwise specificity of peptide signals with hierarchical clustering performed on 350 peptides ( y axis) and 60 patients plus 10 controls ( x axis) with Euclidean distance used as the measure of separation. The order of each patient and peptide is calculated from the distance measure using hierarchical clustering. Classification of all samples was 100% accurate using either linear discriminant analysis or support vector machine (SVM) with leave-one-out cross-validation. Top left: serum from six different cancers with 10 patients in each group (BC, breast cancer, GBM, Glioblastoma multiformae , MM, multiple myeloma, EC, oesophageal cancer, OV, ovarian cancer, LNG, lung cancer) was analysed using the 330,000 peptide microarray. The striking stair-step pattern is because of the clustering algorithm alone. Top right: Sera from six different infectious diseases, with 10 patients in each group except BP, with five patients (Dengue, dengue virus, VF, Coccidioides immitis , BP, B. pertussis , Lyme, Borrelia burgdorferi , WNV, West Nile Virus, TP, T. pallidum and healthy donors (ND) were likewise analysed. Each sample set achieved 100% accuracy using SVM as the classifier and leave-one-out cross-validation. Below left: a plot of log 10 P value ( x axis) versus log 2 fold-change ( y axis) between 10 randomly selected patients at the time of diagnosis with oesophageal cancer (numerator) and 10 otherwise healthy controls (denominator) displays the distribution of significant peptides and the resulting ratios. In all, 562 peptides with P -val <3 × 10 −7 are coloured red, yielding a 0.017% false-positive rate. Lower right is a power plot demonstrating the minimum detectable fold-change (delta, black line, calculated using the command power.t.test() in R) along the x axis. This power plot is reviewed in detail in ref. 30 . The blue bars ( y axis) represent every peptide’s average log2 ratio between 10 oesophageal cancer patients (numerator) and 10 healthy controls (denominator). The red circles indicate the same peptides as in the graph to the left ( P <3 × 10 −7 ). Full size image Statistical analysis of immunosignature performance The immunosignature data in Fig. 2 were analysed using Type I analysis of variance (ANOVA) analysis followed by feature selection using pattern matching to restrict peptides to those with the highest contrast between each disease and all other samples. The 350 peptides shown in Fig. 2 top left (six cancers and normal controls) had ANOVA P values less than or equal to 10 −21 . A 1,000 × permuted t -test (labels between oesophageal cancer and healthy controls were shuffled 1,000 times) gives no P values less than 10 −4 , suggesting that patterns do not arise randomly but are specific to each disease cohort. For comparison, a similar experiment of five different cancer cohorts, 20 persons each, using a printed peptide array of 10,000 random-sequence peptides yielded 100 peptides with P <10 −14 or smaller by ANOVA. The 350 peptide feature intensities displayed in Fig. 2 top right arose from an analysis of six different infectious diseases versus healthy controls. ANOVA yielded 350 peptides with P <10 −22 or smaller. A 1,000 × permuted t -test gave P values >10 −4 . A similar analysis of 45 Valley Fever patients versus 34 controls gave 243 peptides with P <10 −17 . Figure 2 bottom left demonstrates the relationship between array-to-array precision and the associated ability to detect changes between patients with oesophageal cancer and healthy controls. The log 2 ratio across the cohort of eight oesophageal cancer patients versus eight healthy volunteers is plotted on the y axis. Peptides that have higher intensity for the oesophageal cancer patients than controls are plotted above the x axis (positive log 2 ratio), those that are lower in oesophageal patients than controls are below the x axis. The log 10 P value is plotted along the x axis. The red circles indicate those peptides that are significant at P <1 × 10 −6 . Figure 2 lower right is a power plot of the same data. The log 2 ratio is plotted as blue bars extending above the x axis (peptides higher in oesophageal cancer than control) or below the x axis (peptides lower in oesophageal cancer than control). The black curve indicates the minimal detectable fold-change for each of the 330,000 peptides calculated by an a posteriori power analysis that was calculated using a two-sided power test with alpha=0.05, beta=0.20, N =10 per arm, actual s.d. calculated per peptide. The closer the black line is to the x axis, the more precision that peptide has, and the smaller the difference that peptide was able to detect. Peptides on the far right of the power chart indicate those peptides where precision is low and the minimum detectable fold-change is very high. Red circles are the same significant peptides ( P <1 × 10 −6 ) as in the volcano plot on the left. The power plot and volcano plot represent the general performance of the 330,000 peptide microarray, which far exceeds the precision inherent in modern commercial expression microarrays [30] . There are 23,323 informative peptides on the array that contribute to distinguish oesophageal cancer patients from healthy controls. We do not imply that the particular peptide signatures for each condition constitute a diagnostic for that disease; that would require larger cohorts and blinded tests. However, these results indicate that the high-density arrays can produce consistent immunosignatures, an important step in enabling large-scale applications of immunosignaturing. Past work has demonstrated the potential of immunosignature technology as a useful diagnostic for detection of chronic disease and infectious disease, symptomatic [12] , [13] , [16] as well as early [15] . However, the research platform upon which most of this work was based is difficult to produce at volume and low cost and limited in the number and density of peptide features. Here we demonstrate the production, chemical characterization and diagnostic potential of high-density peptide microarrays on a manufacturing platform that can easily be scaled and follows the same kind of cost/volume characteristics and electronics manufacturing. We believe the greatest potential impact of these arrays is enabling regular, comprehensive health monitoring. The number of unique peptides in these arrays makes it feasible to detect and distinguish many different disease signatures simultaneously. The scalability and associated low cost of the process should make it feasible for individuals to monitor their health on a frequent basis, providing the additional advantage of establishing a robust personal health baseline. Using arrays of non-natural peptide sequences designed to evenly represent combinatorial sequence space has the advantage of making the immunosignature platform a universal diagnostic technology. For any new condition, a new format or physical array is not needed; the same data simply need to be analysed in terms of a different reference signature. However, a disadvantage of this approach relative to using peptide sequences from known proteomes is that the signatures cannot be directly ‘read’ back to the original antigen. The identity of the antigen would have to be inferred informatically from the collection of peptides that makes up a signature (see Supplementary Tables 1 and 2 ). The larger number of peptides available in the 330,000 peptide arrays facilitates this process. Obviously, high density, low cost, peptide arrays have many other possible uses besides health monitoring. Peptide arrays have been used to assay kinase activity and inhibitors [23] , [31] , map monoclonal antibodies [32] , identify autoantigens [33] , even bind proteins [34] and cells [35] . The synthesis fidelity and peptide density of these arrays make it feasible to tile the entire human proteome or the proteomes of most human pathogens for studies of autoimmunity or vaccine development [23] , [26] , [36] . Random-sequence arrays have been the starting point for developing synthetic antibodies [34] , [35] , [37] , [38] using branched peptides, and a screening system for identifying antimicrobial peptides [35] . We expect this platform will find many other uses. Lithography-based peptide array synthesis The procedure for synthesis of the arrays is shown schematically in Fig. 3a . The arrays were fabricated to specification by HealthTell Inc. for the studies described here. A 520-nm thermal oxide-coated silicon wafer surface is derivatized with a monolayer of aminosilane to create peptide attachment sites, and Boc-glycine is uniformly attached to the surface. A photoresist containing a photoacid generator is spun on the wafer and exposed through a defined mask (Topan, Santa Clara, CA, USA) to 365-nm light, resulting in the patterned deprotection of Boc-protected amines in specific features on the array. A coupling solution containing a Boc-protected amino acid is then spun on the wafer and coupling takes place only at the deprotected features. The process is repeated to create the desired peptide sequence at each feature. For the arrays described below, a distribution of peptide lengths was intentionally generated averaging 12 amino acids along with individual peptides ranging from 8 to 17 aa. This length distribution was chosen because it is similar to the length distribution of antibody epitopes that range from 5 to 15 aa [39] . The sequence of each peptide was pseudo-randomly generated using an algorithm that minimizes the number of synthetic cycles required, and uses 16 of the 20 natural amino acids, with cysteine, methionine, isoleucine and threonine excluded. As an immunosignature is not based on natural sequence space per se , but instead on a representative and diverse chemical space, it was not necessary to use all amino acids, a fact that simplifies synthesis, reducing the total number of steps to 90 lithography cycles at ~20 min per cycle. Peptide arrays are synthesized with 8-μm features and a 12-μm centre-to-centre spacing in an orange-crate pattern. The 200-mm wafers are diced into 13 75 × 25 mm slides, each with 24 identical arrays of 330,000 distinct peptides (~8 M peptides per slide) The total assay area of each array is 0.49 cm 2 and the 24 assay per slide format allows existing robotics designed for microscope slides and 96-well enzyme-linked immunosorbent assay (ELISA) plates to be used with no modification. Scanning of the slides is performed using commercially available laser scanners. If configured as a single array, the system could produce ~10 M different peptides per standard slide. 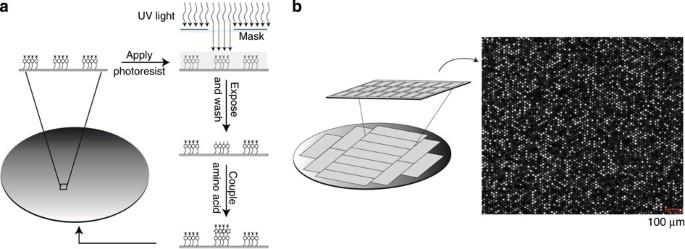Figure 3: Immunosignature array synthesis. (a) Mask-based patterned synthesis of peptides was performed on 200-mm silicon wafers with thermal oxide coating, starting with an aminosilane–glycine monolayer and building peptides through cycles of patterned acid formation in a photoresist removing Boc groups from theN-terminal amines of nascent peptides and coupling of the next amino acid. (b) The wafer is diced into microscope slide-sized regions (75 × 25 mm), each of which contains 24 arrays of 300 and 30,000, 8-μm features. Samples can individually be applied to each array via a commercially available gasket system and scanned on a laser scanner. On the far right is an image of the array (at × 800 magnification) of serum applied to the array and detected with fluorescent secondary antibody. Figure 3: Immunosignature array synthesis. ( a ) Mask-based patterned synthesis of peptides was performed on 200-mm silicon wafers with thermal oxide coating, starting with an aminosilane–glycine monolayer and building peptides through cycles of patterned acid formation in a photoresist removing Boc groups from the N- terminal amines of nascent peptides and coupling of the next amino acid. ( b ) The wafer is diced into microscope slide-sized regions (75 × 25 mm), each of which contains 24 arrays of 300 and 30,000, 8-μm features. Samples can individually be applied to each array via a commercially available gasket system and scanned on a laser scanner. On the far right is an image of the array (at × 800 magnification) of serum applied to the array and detected with fluorescent secondary antibody. Full size image Assay and scanning The 24 assay per slide arrangement enables ELISA-based fluidics systems to be used. Ninety-six-well gaskets and frames were purchased from ArrayIt (Sunnyvale, CA, USA) that enable four slides to be arrayed in a 96-assay format. A Beckman Biomek FX robot with 96 channel head was used to transfer solutions to the individual arrays while an integrated Biotek 405TS plate washer (Biotek, Winooski, VT, USA) was used to wash the arrays between incubation steps. Assay conditions are described in ref. 16 . Briefly, arrays are deprotected to remove Boc protecting groups [40] and blocked in blocking buffer [16] . There was no preprocessing of serum; 1 μl of serum was diluted 5000-fold in sample buffer [16] and 200 μl was then applied to each 330,000 peptide subarray, incubated for 1hr at 23 °C, washed, and then labelled with a fluorescent secondary antibody for human IgG [16] . The BioTek ELx405 plate washer is programmed to wash four separate 24-up arrays four times for five minutes each using incubation buffer. Note that the microarrays are designed to fit into standard laser scanners. The fluorescent intensity at each peptide was measured using an Innoscan 900 1 μm scanner (Innopsys, Chicago, IL, USA) using the 545-nm laser, scanned at 1 μm resolution. Each subarray was scanned and aligned separately, with 24 high-resolution Tagged Image File Format images produced per slide. Quality control The accuracy of the immunosignaturing platform relies on the production of highly reproducible arrays of peptides that are both chemically consistent from array to array and are accessible for antibody binding. Immunosignature and other applications depend on the chemical fidelity of peptide synthesis as well as the density of peptides at each feature. A quantitative analysis of the chemical composition of peptide features on immunosignature arrays is given in Fig. 1 using high-resolution mass spectrometry performed by NextVal Inc. (San Diego, CA, USA). In Fig. 1a , multiple copies of three different epitope sequences were synthesized in a randomly distributed manner and probed with the appropriate monoclonal antibodies. Each monoclonal bound its own epitope on the array at least 100-fold higher than either of the other two. The current masks enable thousands of versions of the linear epitopes for each of nine different commercially available monoclonal antibodies HA [HA tag, sequence: YPYDVPDYA, Rockland Antibodies, Rockland, MD], Ab1 [Hu TP53, sequence TFRHSVVV, aa210–218, Clonetech, Palo Alto, CA], Ab8 [Hu TP53, sequence TFSDLWKLLPE, aa18–28, LabVision/Thermo, Anthem AZ], Cdc2 [Hu Cyclin Dependent Kinase 1, sequence: TPNNEVWPEVE, aa 221–231, Abcam, Cambridge, UK], LNKB2 [Hu Interleukin2,sequence: KPLEEVLNL, aa64-72, Santa Cruz Biotech, Dallas TX], DM1A [Hu Tubulin alpha subunit, sequence: AALEKDYEEVGV, aa 73–85, Life Technologies, Carlsbad, CA], HSV [HSV1, sequence: QPELAPEDPED, aa379–389, Abcam, Cambridge, UK], 4C1 [hTSHr Hu Insulin receptor, sequence: QAFDSHY, aa379–385, Santa Cruz Biotech], A10 [hTSHr Hu Insulin receptor, sequence: EEDFRVT, aa33–40, Santa Cruz Biotech] to appear at scattered locations across each array. The epitopes appear as written or with random surrounding sequence. Human subjects Human serum was used to test the microarrays for the ability to produce accurate and reproducible immunosignatures, as in refs 13 , 16 . Retrospective collections of serum or plasma work as well as newly drawn samples [8] . The infectious disease samples were purchased from SeraCare Life Sciences (Milford, MA, USA) and were consented upon collection. Cancer samples were acquired from collaborators and were consented upon collection through the institute’s own IRB. All samples were anonymized before receipt at ASU via Institutional Review Board (IRB) no. 0912004625, ‘Profiling Biological Sera for Unique Antibody Signatures’ (approved by the Western Institutional Review Board, Olympia, WA, USA). Healthy volunteers were recruited at Arizona State University through the aforementioned IRB. How to cite this article: Legutki, J. B. et al. Scalable high-density peptide arrays for comprehensive health monitoring. Nat. Commun. 4:4785 doi: 10.1038/ncomms5785 (2014).